Efficient and tunable white-light emission of metal–organic frameworks by iridium-complex encapsulation Metal–organic frameworks (MOFs) are well known for their tunable structure and porosity. Many studies have shown they are promising for various important applications, for which their performance can be further enhanced by encapsulating functional species, such as luminescent guest molecules, within the frameworks. Although numerous MOFs are luminescent, very few emit white light and their quantum yield is usually low. Here we report a strategy to achieve efficient white-light emission by encapsulating an iridium complex in the MOF cavity. A mesoporous blue-emitting MOF is prepared as host to encapsulate a yellow-emitting iridium complex, [Ir(ppy) 2 (bpy)] + . The resultant composites emit bright white light with good colour quality (for example, Commission International de I’Eclairage coordinates, colour-rendering index and correlated colour temperature of (0.31, 0.33), 84.5 and 5409 K, respectively), and high quantum yield up to 115 °C. This strategy may open new perspectives for developing high-performance energy-saving solid-state lighting materials. Solid-state light-emitting-diode (LED) materials have been extensively investigated in the recent years because of their potential applications in lighting and displays [1] , [2] . Currently, mercury-containing fluorescent lighting is one of the most widely used white-light sources, which relies on the emission of mercury vapour to excite semiconductor phosphors and to achieve white composite photoluminescence (PL) [3] . However, the extensive use of mercury raises various environmental concerns. Thus tremendous efforts have been dedicated to search for environmentally more friendly, safer and more energy efficient white phosphor materials for use in the white LEDs (WLEDs) [4] , [5] , [6] , [7] , [8] , [9] , [10] , [11] , including hybrid inorganic materials [4] , [5] , [10] , [11] , rare-earth metal-doped zeolites [6] , organic compounds [7] , nanomaterials [8] and metal complexes [9] . Three types of white phosphor materials are commonly used in phosphor-based methods to generate white light, including (i) monochromatic emitters that emit in the entire visible spectrum, (ii) dichromatic emitters that blend blue and yellow light and (iii) trichromatic emitters that combine red, green and blue lights. Among them, dichromatic and trichromatic approaches have been the main focus because of their finer colour-rendering properties and higher luminescent efficiency [12] . Metal−organic frameworks (MOFs) composed of metal ions and multitopic organic ligands are a new family of hybrid inorganic–organic porous materials, and have received tremendous attention in the past two decades [13] , [14] , [15] . Benefiting from uniform but tunable cavities, tailorable chemistry and high porosity, MOFs have become promising candidates for many important applications such as chemical separation [16] , gas storage [17] , catalysis [18] , drug delivery [19] and optical sensing/detection [20] . MOF materials possess unique advantages for luminescence-based applications primarily because of their capability of incorporating light-emissive building blocks at both metal centres and organic ligands. This allows efficient modulation of luminescent properties. In addition, permanent porosity in these structures permits the accommodation of guest molecules within their frameworks, offering another degree of tunability in their emission properties [21] . Through judicious choice of metal centres and organic linkers, a large number of luminescent MOFs have been synthesized (accounting for >10% of the total number of reported MOFs) and their possible applications in fluorescent sensors, nonlinear optics, photocatalysis and biomedical imaging have been evaluated [22] . On the other hand, it remains a great challenge to produce high-performance white-emitting MOF materials suitable for solid-state lighting applications. To date, only a few examples of direct white-light-emitting MOFs are realized [23] , [24] , [25] , [26] . Doping the framework structures by rare metals (for example, Eu 3+ , Tb 3+ and Dy 3+ ) at various concentrations may lead to white light [12] , [27] , [28] , [29] , but at low quantum yield [12] . Thus, it is essential to develop an effective method to obtain highly efficient, white-light-emitting MOF materials. Herein, we introduce a new strategy to achieve high quantum yield white light by encapsulating a yellow-emitting Ir III complex in the cavity of a blue-emitting MOF. Ir III complexes are well known for their high PL efficiency, relatively short lifetimes and emissive light variety [30] . Large-pore MOF structures with tunable pore sizes (up to 9.8 nm (ref. 31 )) may be constructed by suitable choice of organic ligands of various length which will ensure the entrapment of Ir III complexes in large quantity. Thus, it may be anticipated that a successful encapsulation of yellow-emitting Ir III complex in a blue-emitting MOF will not only produce white light, but also generate high quantum yield, because the aggregation of Ir III complexes can be effectively prevented and their oscillation may also be effectively constrained when confined into the MOF pores [32] . A cationic Ir III complex, [Ir(ppy) 2 (bpy)] + (Hppy=2-phenylpyridine, bpy=2,2′-bipyridine), was selected in this study as an encapsulate for its relatively small size which allows easy access to the MOF pores. Hexadentate carboxylate triazine ligand, 2,4,6-tris(2,5-dicarboxylphenylamino)-1,3,5-triazine (H 6 TATPT, Supplementary Fig. S1 ) was chosen as the organic building block to construct highly porous blue-light-emitting MOF, based on the following considerations: (i) it has a suitable length for building MOF structures with desired pore diameters [33] , [34] , (ii) it offers multiple metal binding modes and (iii) it emits at 490 nm which will likely result in a blue-emitting MOF material. Cadmium ion was selected as metal centre because d 10 metal ions not only possess various coordination numbers and geometries, but also exhibit photoactive capability when bound to functional ligands [35] . With TATPT and Cd 2+ , we successfully prepared a three-dimensional (3D) mesoporous blue-emitting anionic MOF, [(CH 3 ) 2 NH 2 ] 15 [(Cd 2 Cl) 3 (TATPT) 4 ]·12DMF·18H 2 O ( 1 ) which contains two types of cages with the dimensions of approximate 2 and 3 nm. Compound 1 emits bright blue light ( λ em =425 nm) attributed to the emissive organic TATPT linker. [Ir(ppy) 2 (bpy)] + was successfully loaded into the pores of 1 to form [Ir(ppy) 2 (bpy)] + @ 1 at various concentrations. The new composite emitter generates bright white light when excited at 370 nm with a quantum yield as high as 20.4%. This value is the highest among all white-light-emitting MOF materials reported to date [12] , [23] , [24] , [25] , [26] , [27] , [28] , [29] and is approaching the level of the best inorganic–organic hybrid semiconductor bulk materials [36] . At an [Ir(ppy) 2 (bpy)] + concentration of 3.5 wt%, the Commission International de I’Eclairage (CIE) coordinates, colour-rendering index (CRI) and correlated colour temperature (CCT) values were calculated to be (0.31, 0.33), 80 and 5900 K, respectively. A WLED assembly built on an ultraviolet LED chip (InGaAsN, 370 nm) and an [Ir(ppy) 2 (bpy)] + @ 1 sample at 3.8 wt% of Ir-complex yielded (0.30, 0.35), 84.5 and 5409 K for CIE, CRI and CCT, respectively. X-ray diffraction analysis of compound 1 Compound 1 was synthesized by reacting H 6 TATPT and CdCl 2 ·2.5H 2 O (1:1 molar ratio) in a N,N-dimethylformamide (DMF)/MeOH solvent mixture heated at 120 °C for 2 days. The reaction produced colourless crystals with polyhedral morphology ( Supplementary Fig. S2 ). The phase purity of 1 was confirmed by powder X-ray diffraction (PXRD) analysis. The formula of 1 was obtained by single-crystal X-ray diffraction, elemental analysis (EA), thermogravimetric analysis (TGA) and by taking into account charge balance considerations. The protonated [(CH 3 ) 2 NH 2 ] + is a result of decomposition of DMF [37] . Single-crystal X-ray diffraction analysis reveals that 1 is a 3D non-interpenetrated framework. It crystallizes in cubic space group Fm -3 m ( Supplementary Table S1 ). The asymmetric unit of 1 contains one crystallographically independent cadmium ion, one chlorine ion and one-sixth of TATPT ligand. Other disordered cations and guest molecules are not crystallographically well defined. Compound 1 is built on a cuboid Cd 2 ( μ 2 -Cl)(CO 2 ) 8 secondary building unit (SBU). In this SBU, the two Cd atoms are nine-coordinated by a μ 2 -Cl and eight carboxylate oxygen atoms from four TATPT ligands in enneahedral geometry ( Supplementary Fig. S3a ). The μ 2 -Cl atom connects the two Cd atoms lying at the centre of the rectangular parallelepiped. The bond lengths of Cd–O carboxylate (2.285–2.646 Å) are within the normal range of those reported cadmium–carboxylate compounds and the bond lengths of Cd–Cl (2.699 Å) are close to the reported cadmium–chlorine compounds. Each SBU is eight-coordinated to four TATPT ligands, and each TATPT is six-connected to three SBUs ( Supplementary Fig. S3b ) to form a truncated tetrahedron [38] ( Fig. 1a ), in which all six vertices are occupied by the SBUs, and four of the hexagonal faces are held by TATPT ligands. The dimension of the truncated tetrahedral cage is 19.2 × 16.7 × 16.3 Å 3 (measured between opposite atoms and van der Waals radii of the atoms are not taken into account) and the size of windows is about 11 × 11 Å 2 . Eight such truncated tetrahedrons occupy the eight vertices of a cube, resulting in a mesoporous truncated octahedron [38] ( Fig. 1b ) through corner sharing. The dimensions of this truncated octahedron are 27.2 × 23.1 × 27.2 Å 3 with a window size of ~15.5 × 15.5 Å 2 . The truncated octahedra propagate to form a three-dimensional non-interpenetrated extended open network ( Fig. 1c and Supplementary Fig. S3 ). The pore structure can also be viewed as three intersecting1D channels with a window size of 15.5 × 15.5 Å 2 . From the topological point of view, each of the Cd 2 ( μ 2 -Cl)(CO 2 ) 8 SBU acts as a four-connected node and every TATPT ligand serves as a three-connected node, thus the framework can be described as a binodal (3,4)-connected 3D network with tbo topology (Schläfli symbol (6 2 .8 2 .10 2 ) 3 (6 3 ) 4 ) ( Fig. 1d ). The solvent molecules and [(CH 3 ) 2 NH 2 ] + cations reside in the channels. The effective free volume of 1 , calculated by PLATON software [39] , is 67.8% of the crystal volume (38,769.5 Å 3 of the 57,186.8 Å unit cell volumes), upon removal of the guest molecules. 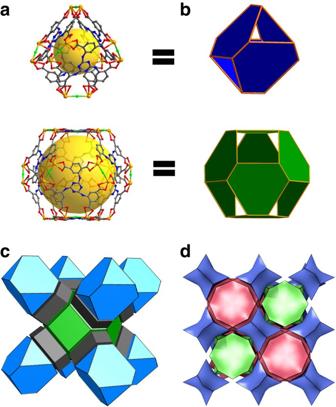Figure 1: Structure of1determined by single-crystal XRD. (a) Ball and stick representations of the truncated tetrahedral and truncated octahedral cages, the yellow spheres represent the void inside the cages. (b) Polyhedral presentation ofa. (c) The 3D polyhedral structure of1. (d) The (3,4)-connected augmented net (top) as a natural tiling. Figure 1: Structure of 1 determined by single-crystal XRD. ( a ) Ball and stick representations of the truncated tetrahedral and truncated octahedral cages, the yellow spheres represent the void inside the cages. ( b ) Polyhedral presentation of a . ( c ) The 3D polyhedral structure of 1 . ( d ) The (3,4)-connected augmented net (top) as a natural tiling. Full size image TGA and transition metal ion exchange experiments Overall, the framework structure is anionic with H 2 O molecule, (CH 3 ) 2 NH 2 + cations as well as DMF residing in the channels, as determined by EA, TGA and by the consideration of charge balance. The TGA data ( Supplementary Fig. S4 ) reveal that the first weight loss corresponds to the loss of solvent and water molecules (20.3 wt%). The desolvated framework remains stable until ~210 °C ( Supplementary Fig. S4 ). The decomposition of the framework began to take place at this temperature. The final residue is CdO (observed 16.0%, calculated 15.1%). Furthermore, transition metal cation exchange experiments were performed by soaking samples of 1 in solutions of Cu(NO 3 ) 2 ·3H 2 O, Co(NO 3 ) 2 ·6H 2 O, Ni(NO 3 ) 2 ·6H 2 O and Zn(NO 3 ) 2 ·6H 2 O in DMF solvent, respectively. After a few days the colour of the solid changed from colourless to teal, red and light green, for Cu 2+ , Co 2+ and Ni 2+ , respectively ( Supplementary Fig. S5 ). For Zn(NO 3 ) 2 , no colour change was observed. A PXRD comparison of 1 before and after exchange experiments indicates that the integrity of 1 is retained after transition metal cation exchange uptake ( Supplementary Fig. S6 ). The successful exchange of (CH 3 ) 2 NH 2 + with transition metal cations was confirmed by 1 H NMR spectroscopic studies after cation exchange experiments ( Supplementary Fig. S7 ). The products were characterized by Inductively coupled plasma (ICP) spectroscopy ( Supplementary Table S2 ) and the results show that approximately 0.46 Cu II , 0.37 Co II , 0.26 Ni II and 0.28 Zn II per formula was impregnated into the framework. PL measurements of H 6 TATPT and compound 1 The emission spectra of the H 6 TATPT ligand, and compound 1 in powder form were measured at room temperature and displayed in Supplementary Fig. S8 . The free H 6 TATPT ligand exhibits a weak emission at 490 nm under the excitation at 370 nm, which is due presumably to the π → π * transition of the intraligands [40] . Upon excitation at the same wavelength, compound 1 shows significantly enhanced bright blue light emission with an emission maximum at 425 nm ( Supplementary Fig. S9 ) [41] . Compared with the free organic linker, the large enhancement of emission intensity and strong blue shift (about 65 nm) of the emission in 1 may be attributed to metal-to-ligand charge transfer (MLCT) and the coordination effects of the ligand to Cd (II) cations, which increases the ligand conformational rigidity and reduces the non-radiative decay [42] . The CIE coordinates for the blue emission of compound 1 was calculated to be (0.175, 0.145), close to that of saturated blue emitter with CIE coordinates of (0.14, 0.08) [43] . The quantum yield of compound 1 was measured under λ ex =370 nm at room temperature and a value of 15.1% was obtained. These data demonstrate that compound 1 is an efficient blue-light emitter [44] . Encapsulating [Ir(ppy) 2 (bpy)] + in compound 1 Primary Ir III complex, [Ir(ppy) 2 (bpy)] + (with a counter ion [PF 6 ] − ), was selected as the encapsulant [45] . With a molecular size of ~10 × 11 Å 2 which is smaller than the aperture of the pore windows of compound 1 , the complex can enter the pores readily. The [Ir(ppy) 2 (bpy)][PF 6 ] complex was synthesized according to the reported procedure [46] and its structure is shown in Fig. 2 . The emission spectrum of [Ir(ppy) 2 (bpy)][PF 6 ] was measured in DMF solution at room temperature and plotted in Supplementary Fig. S10 . From the emission spectrum it is clear that when excited at 370 nm, [Ir(ppy) 2 (bpy)][PF 6 ] emits yellow light with broad and structureless emission at 570 nm, indicating a predominant 3 MLCT or 3 LLCT character [47] , [48] . 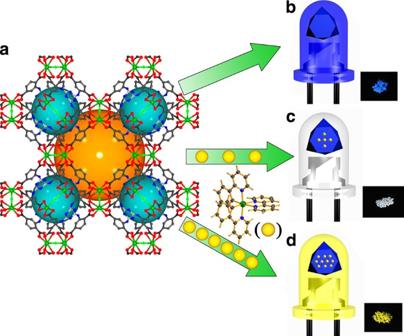Figure 2: Scheme of the encapsulation of [Ir(ppy)2(bpy)]+in compound1. (a) Ball and stick representations of the 3D structure of1, the orange and dark cyan spheres represent the void inside the cages. (b) When radiated under a standard laboratory ultraviolet lamp (365 nm), compound1emits bright blue light. (c,d) [Ir(ppy)2(bpy)]+- encapsulated samples [Ir(ppy)2(bpy)]+@1emit bright white (3.5 wt%) and yellow (8.8 wt%) light, respectively, using the same 365 nm ultraviolet lamp. Figure 2: Scheme of the encapsulation of [Ir(ppy) 2 (bpy)] + in compound 1 . ( a ) Ball and stick representations of the 3D structure of 1 , the orange and dark cyan spheres represent the void inside the cages. ( b ) When radiated under a standard laboratory ultraviolet lamp (365 nm), compound 1 emits bright blue light. ( c , d ) [Ir(ppy) 2 (bpy)] + - encapsulated samples [Ir(ppy) 2 (bpy)] + @ 1 emit bright white (3.5 wt%) and yellow (8.8 wt%) light, respectively, using the same 365 nm ultraviolet lamp. Full size image In an initial attempt, powder samples of 1 were immersed into DMF solutions of [Ir(ppy) 2 (bpy)] + (10 −4 mol·l −1 ) in duplicate. After 7 and 10 days, both soaked samples were removed from the solution. An obvious colour change from colourless to light yellow was observed, indicative of a successful encapsulation of [Ir(ppy) 2 (bpy)] + into the framework of compound 1 . As evidenced from the PXRD data, the [Ir(ppy) 2 (bpy)] + @ 1 samples maintain their crystallinity ( Supplementary Fig. S11 ). The concentrations of encapsulated [Ir(ppy) 2 (bpy)] + were measured by ICP experiment. The results show that ~7.5 wt% and ~8.8 wt% [Ir(ppy) 2 (bpy)] + were embedded, respectively, with respect to Cd. PL spectra were collected on both [Ir(ppy) 2 (bpy)] + @ 1 samples. As shown in Fig. 3 (yellow and orange curves), the PL spectra of both samples exhibit two emission maxima at ~425 and ~530 nm, respectively, when irradiated at 370 nm. The emission at 425 nm is attributed to MLCT in 1 whereas the emission at 530 nm presumably originates from [Ir(ppy) 2 (bpy)] + . However, in comparison with the emission of free [Ir(ppy) 2 (bpy)] + , there is an obvious blue shift (about 40 nm) in the emission spectra of the [Ir(ppy) 2 (bpy)] + @ 1 composites. A possible explanation for such large blue shift is that the confinement of [Ir(ppy) 2 (bpy)] + within the pores of 1 leads to a phenomenon very similar to a ‘rigidochromic effect’ reported and explained previously on similar metal complexes [49] , [50] , [51] . The corresponding CIE coordinates were calculated and the values are (0.37, 0.47) and (0.40, 0.50) for 7.5 wt% and 8.8 wt% encapsulated samples, respectively, at an excitation wavelength ( λ ex ) of 370 nm. The quantum yield of the 8.8 wt% [Ir(ppy) 2 (bpy)] + @ 1 sample was measured at room temperature. A value of 28.7% was achieved at λ ex =370 nm. The photograph of its emission is shown in Fig. 2d , Supplementary Fig. S12c and Supplementary Fig. S13 , excited at 365 nm using an ultraviolet lamp. Another interesting phenomenon observed in the PL spectra is that the intensity of the 530 nm emission is higher for the 8.8 wt% than for the 7.5 wt% encapsulated sample, whereas the intensity of 425 nm emission is similar for the two samples. This is another evidence that the 530 nm emission is due to [Ir(ppy) 2 (bpy)] + . 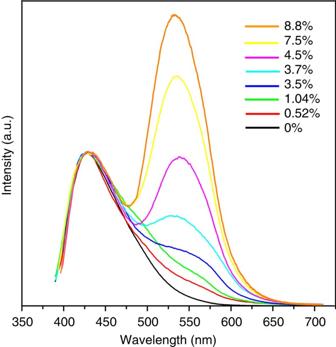Figure 3: PL spectra of 1 and [Ir(ppy)2(bpy)]+encapsulated1. Room temperature emission spectra of1and [Ir(ppy)2(bpy)]+@1with different concentration of [Ir(ppy)2(bpy)]+: black, emission spectrum of1; red, 0.52 wt% [Ir(ppy)2(bpy)]+at1; green, 1.04 wt%; blue, 3.5 wt%; cyan, 3.7 wt%; pink, 4.5 wt%; yellow, 7.5 wt%; orange, 8.8 wt%. All measurements were performed on solid samples at an excitation wavelength (λex) of 370 nm. Figure 3: PL spectra of 1 and [Ir(ppy) 2 (bpy)] + encapsulated 1 . Room temperature emission spectra of 1 and [Ir(ppy) 2 (bpy)] + @ 1 with different concentration of [Ir(ppy) 2 (bpy)] + : black, emission spectrum of 1 ; red, 0.52 wt% [Ir(ppy) 2 (bpy)] + at 1 ; green, 1.04 wt%; blue, 3.5 wt%; cyan, 3.7 wt%; pink, 4.5 wt%; yellow, 7.5 wt%; orange, 8.8 wt%. All measurements were performed on solid samples at an excitation wavelength ( λ ex ) of 370 nm. Full size image Fabrication of WLEDs of [Ir(ppy) 2 (bpy)] + @1 composite To obtain white-light emission, a more balanced distribution of the two emissions is needed. This can be accomplished by reducing the amount of [Ir(ppy) 2 (bpy)] + in compound 1 . The corresponding PL spectra of [Ir(ppy) 2 (bpy)] + encapsulated samples at different concentrations were collected and plotted in Fig. 3 . The PL spectra show that the intensity of the emission at 530 nm decreases monotonically as the [Ir(ppy) 2 (bpy)] + amount decreases. White-light emission was achieved as the concentration of Ir complex was adjusted from 1.04 wt% to 3.7 wt% (see Fig. 4 , and Supplementary Table S3 ). The optimal concentration for the white light was found to be 3.5 wt%, with CIE coordinates of (0.31, 0.33). This is very close to those of the pure white light (0.33, 0.33). Other related colour parameters, including the CCT and CRI, were also estimated. At this concentration, these values are ~80 and ~5,900 K, respectively. The quantum yield was measured and a value up to 20.4% was obtained ( λ ex =370 nm) for this sample. This value is the highest among all reported white-light-emitting MOFs [12] , [23] , [24] , [25] , [26] , [27] , [28] , [29] to this date ( Supplementary Table S4 ), and is approaching that of the best inorganic–organic hybrid semiconductor white-light emitters [36] . Photographs showing white-light emission of a 3.5 wt% [Ir(ppy) 2 (bpy)] + @ 1 sample under radiation at 365 nm (ultraviolet lamp) are given in Fig. 2b and Supplementary Fig. S12 . 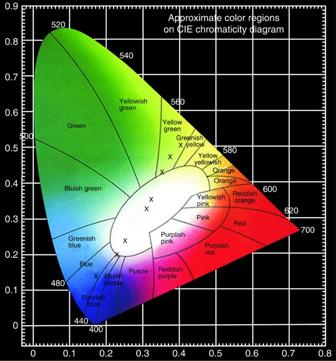Figure 4: CIE-1931 chromaticity diagram. The CIE coordinates (marked by the crosses) for1and [Ir(ppy)2(bpy)]+@1at various concentrations of [Ir(ppy)2(bpy)] (λex=370 nm). Figure 4: CIE-1931 chromaticity diagram. The CIE coordinates (marked by the crosses) for 1 and [Ir(ppy) 2 (bpy)] + @ 1 at various concentrations of [Ir(ppy) 2 (bpy)] ( λ ex =370 nm). Full size image Clearly, the observed broad emission of [Ir(ppy) 2 (bpy)] + @ 1 is simply a combination of the two independent emissive component, [Ir(ppy) 2 (bpy)] + and 1 . Such an additive behaviour is possible when there is essentially no energy and electron/charge transfer between the two species. This is evident from the absorption and emission spectra of the individual components [52] ( Supplementary Figs S14 and S15 ) and the fact that the second emission peak of [Ir(ppy) 2 (bpy)] + @ 1 is independent from the first and is a monotonic function of Ir concentration ( Fig. 3 ). To further verify this, we have carried out lifetime measurements on 1 and [Ir(ppy) 2 (bpy)] + @ 1 at λ ex =370 nm and λ em =425 nm by time-correlated single photon counting. The results show that compound 1 exhibits single-exponential decay behaviour with a lifetime of ~0.84 ns ( Supplementary Fig. S16 ). The lifetime is 0.77 and 0.75 ns for the 3.5 and 8.8 wt% of [Ir(ppy) 2 (bpy)] + @ 1 , respectively). These data indicate that the lifetimes of 1 and [Ir(ppy) 2 (bpy)] + encapsulated samples remain little affected, and thus, confirming that there is no energy transfer between the two components ( [Ir(ppy) 2 (bpy)] + and 1 ) [53] . To evaluate the temperature effect on the emission, PL spectra ( Supplementary Fig. S17 ) and quantum yield ( Supplementary Table S5 ) of [Ir(ppy) 2 (bpy)] + @ 1 were collected at various temperatures. As shown in Supplementary Fig. S17 , the intensity of the yellow emission (530 nm) is essentially unaffected over the entire temperature range investigated. For blue emission (425 nm), a very small change is observed below 115 °C. Above this temperature, the emission intensity and consequently, quantum yield, are reduced considerably. At 150 °C, a ~40% loss is observed ( Supplementary Fig. S17 ). This is due to the partial degradation of the MOF framework upon heating at high temperatures. Thus, [Ir(ppy) 2 (bpy)] + @ 1 is relatively stable only below 115 °C. WLED assemblies using this material were fabricated by two methods. The first one employed a commercially available ultraviolet LED (similar to the reported procedure [36] ) and an [Ir(ppy) 2 (bpy)] + @ 1 sample (Ir complex: 3.5 wt%) as phosphor. The resultant WLED exhibits bright white light at an applied voltage of 3.8 V (see Fig. 5 ). The second WLED was made by an InGaAsN chip (370 nm) and an [Ir(ppy) 2 (bpy)] + @ 1 sample at an [Ir(ppy) 2 (bpy)] + concentration of 3.8 wt% ( Supplementary Fig. S18 ). The latter yielded a CIE, CCT and CRI values of (0.30, 0.35), 84.5 and 5409 K ( Supplementary Table S6 ), respectively. On the basis of these results, it is clear that the [Ir(ppy) 2 (bpy)] + @ 1 materials not only have potential for practical lighting applications, but more importantly, this method of encapsulation of a luminescence-active molecular complex into a luminescent MOF to generate white light and to systematically tune the emission quality also represents a new approach to fabricate WLEDs with superior performance. 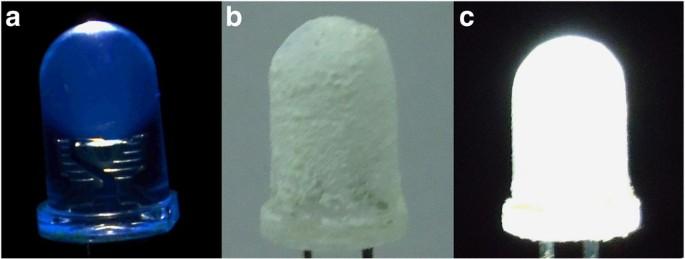Figure 5: Photographs of the LEDs. (a) An illuminating 3 mm reference ultraviolet LED (turned-on emission has a blue tinge). (b) The same LED coated with a thin layer of sample of 3.5 wt% [Ir(ppy)2(bpy)]+@1(not turned on). (c) The coated LED was turned on and illuminates bright white light. Figure 5: Photographs of the LEDs. ( a ) An illuminating 3 mm reference ultraviolet LED (turned-on emission has a blue tinge). ( b ) The same LED coated with a thin layer of sample of 3.5 wt% [Ir(ppy) 2 (bpy)] + @ 1 (not turned on). ( c ) The coated LED was turned on and illuminates bright white light. Full size image PL of Eu 3+ and Tb 3+ co-doped emitters Rare-earth ions (for example, Eu 3+ , Tb 3+ and Dy 3+ ) have been commonly used as dopants to obtain white-light emission. To evaluate their effect in 1 , the samples of white-emitting Eu 3+ and Tb 3+ co-doped 1 were prepared ( Supplementary Fig. S19 ) and their luminescent properties were studied. Under the excitation at 370 nm, the MOF emission colour was fine-tuned to white by soaking 1 in DMF solutions containing nitrate salts of Eu 3+ and Tb 3+ in a molar ratio of 1:2. The corresponding CIE coordinates for this sample is (0.36, 0.32), approaching the coordinates of pure white light. 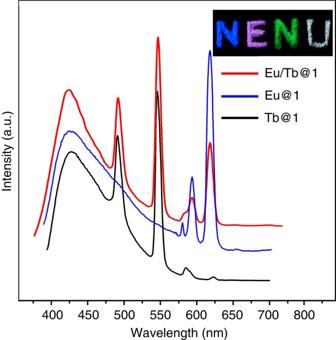Figure 6: PL spectra and optical photographs of lanthanide(III)-doped 1. Room temperature PL spectra of lanthanide(III)-doped1in the solid state upon excitation at 370 nm: black, Tb-doped1; blue, Eu-doped1; red, Eu- and Tb co-doped1.The insets are the optical photographs of1, Eu@1, Tb@1and Eu/Tb@1excited under 365 nm ultraviolet lamps, corresponding to the letters N, E, N and U, respectively. Figure 6 shows photographs of the co-doped samples excited by a standard laboratory ultraviolet lamp (365 nm). The PL spectra of the co-doped samples were also collected under excitation at 370 nm ( Fig. 6 ). These spectra feature a broad emission peak centred at 425 nm and several narrow-band emission peaks at 492, 545, 594 and 618 nm. The broad emission at 425 nm can be attributed to MLCT in 1 . The peaks at 492 and 545 nm are characteristic emissions of Tb cation. The maximal intensities at 594 and 618 nm are corresponding to the emissions of Eu cation. The white-light-emission quantum yield of this sample was measured at room temperature under λ ex =370 nm. A value of 11.3% was obtained which is significantly lower than that of Ir III encapsulated 1 , assuming that the energy migrates through the same electronic levels located in the MOF structure to the doped lanthanide ions [54] . This result indicates that Ir III -complex encapsulating method is likely a more effective approach to obtain high-efficient white-light-emitting MOF materials. On the other hand, introduction of Eu 3+ or Tb 3+ ions into 1 can lead to red and green light emissions. The corresponding PL spectra and the corresponding optical photographs are also given in Fig. 6 . Figure 6: PL spectra and optical photographs of lanthanide(III)-doped 1. Room temperature PL spectra of lanthanide(III)-doped 1 in the solid state upon excitation at 370 nm: black, Tb-doped 1 ; blue, Eu-doped 1 ; red, Eu- and Tb co-doped 1 .The insets are the optical photographs of 1 , Eu@ 1 , Tb@ 1 and Eu/Tb@ 1 excited under 365 nm ultraviolet lamps, corresponding to the letters N, E, N and U, respectively. Full size image In this study, we have demonstrated that encapsulating an Ir III complex cation in the pores of an anionic MOF structure represents a convenient and efficient route to achieve white-light emission with high quantum yield and optimized colour quality. H 6 TATPT was chosen as organic building block in the MOF synthesis, not only for its suitable length [37] , [38] but also for its blue emission which was retained in the resultant framework. A cationic yellow-emitting Ir III complex, [Ir(ppy) 2 (bpy)] + , was selected as the encapsulant based on the consideration of pore size and its complementary yellow emission. [Ir(ppy) 2 (bpy)] + was successfully introduced in the pore of the MOF host via encapsulating experiments. The encapsulated amount can easily be controlled and fine-tuned by varying exposure time and concentration. At an [Ir(ppy) 2 (bpy)] + concentration of 3.5 wt%, high-quality white light was obtained and the resultant material possesses CIE coordinates (0.31, 0.33) that are very close to those of pure white light and good colour quality (CRI ~80 and CCT ~5900 K). In addition, this material also has the highest emission quantum yield (up to 20.4%) compared with all MOFs reported to date [12] , [27] , [28] , [29] , [30] , [31] , [32] , [33] . The WLED assembly using an InGaAsN ultraviolet chip and this material can readily be fabricated. The CIE, CCT and CRI values are (0.30, 0.35), 84.5 and 5409 K, respectively, at a concentration of 3.8 wt% of Ir complex. Eu 3+ and Tb 3+ co-doped samples (Tb/Eu@ 1 ) were also examined on their emission properties. In summary, we have illustrated a judicious design strategy to generate white light by combining the independent emissions of the two components, namely blue emission from the MOF and yellow emission from the Ir complex. The strategy here is essentially the same as the RGB (red, green and blue) combination used in WLED industry to produce white light. We have demonstrated this in a well-controlled manner. We believe that this novel approach opens a new perspective for the development of high performance white phosphors. The new strategy, benefiting from a large number of available luminescent MOF matrix materials and a variety of highly fluorescent metal cationic complexes, offers a great flexibility and very many options in rational selection of matching MOF matrix and metal-complex encapsulate, which, in turn, will facilitate the development of high performance white phosphors with systematically tunable emission properties and greatly enhance quantum efficiency. Materials and measurements All reagents and solvents for the syntheses were purchased from commercial sources and used as received, except H 6 TATPT. ICP spectroscopy was conducted on Agilent 7500a Inductively Coupled Plasma Mass Spectrometry (ICP-MS 7500). PXRD patterns were recorded on a Siemens D5005 diffractometer with Cu K α ( λ =1.5418 Å) radiation in the range 3–50°. EAs (C, H and N) were performed on a Perkin-Elmer 240C elemental analyzer. Solvent 1 H NMR spectra were measured on BrukerAvance 500 MHz with tetramethylsilane as the internal standard. TGA experiments were performed on a Perkin-Elmer TGA 7 analyzer heated from 50 to 800 °C under nitrogen gas atmosphere with a heating rate of 10 °C·min −1 . The emission spectra were recorded using the F-7000 FL spectrophotometer. The PL quantum yields were measured using Hamamatsu multichannel analyzer c10027. Synthesis of ligand H 6 TATPT Cyanuric chloride (1.84 g, 0.01 mol) was added to 150 ml H 2 O and then was stirred at 0 °C for 30 min. After that a mixture of 2-aminoterephthalic acid (1.81 g, 0.01 mol) and NaOH (1 g, 0.025 mol) was added dropwise into the above solution and stirred at<5 °C for 1.5 h. Then 2-aminoterephthalic acid (3.62 g, 0.02 mol) sodium hydroxide solution was added and the reaction mixture was allowed to warm to room temperature. After string at room temperature for 2 h, the mixture was heated slowly to boiling and refluxed for 3 h. During this period, the pH of the mixture was maintained between 10 and 11 by the addition of sodium hydroxide solution. After cooling, the cloudy solution was filtered and the volume was increased to approximated 500 ml by adding 300 ml of water. The solution was acidified with concentrated hydrochloric acid whereupon a crystalline solid precipitated out. The mixture was allowed to cool to room temperature and filtered. After washing thoroughly with cold water, the product was dried in a vacuum oven and the yield was about 90%. 1 H NMR ([D6]DMSO, 400 MHz): δ =8.12 (3H), 8.47 (6H), 9.67 (3H) and 13.0 (6H) ppm. See Supplementary Figs S20 and S21 for high-resolution mass spectrometry and 13 C-NMR data. The structure of H 6 TATPT differs from H 6 TDPAT reported previously in that the carboxylate groups are at 2,5 rather than 3,5 positions [55] . Synthesis of compound 1 A mixture of CdCl 2 (0.10 mmol), H 6 TATPT (0.12 mmol) and 6 ml of DMF/CH 3 OH (1:1) was stirred for 10 min. The mixture was then transferred to and, sealed in, a Teflon reactor (18 ml) and heated at 120 °C for 48 h. After that, the mixture was cooled to room temperature at 5 °C·h −1 . Colourless crystals of 1 were obtained (72.8% yield based on TATPT). EA (%) calculated for [(CH 3 ) 2 NH 2 ] 15 [(Cd 2 Cl) 3 (TATPT) 4 ]·12DMF·18H 2 O (C 174 H 288 N 51 O 78 Cl 3 Cd 6 ): C, 40.71; H, 5.60; N, 13.93; found: C, 40.68; H, 5.62; N, 13.88. Single-crystal X-ray diffraction study Single-crystal X-ray diffraction data for 1 were recorded on a Bruker Apex CCD II area-detector diffractometer with graphite-monochromated Mo Kα radiation ( λ =0.71073 Å) at 293 K. Absorption corrections were applied using multi-scan technique. Their structures were solved by direct method of SHELXS-97 and refined by full-matrix least-square techniques using the SHELXL-97 program. Because guest solvent molecules in channels were highly disordered and could not be modelled properly, thus the SQUEEZE routine of PLATON was applied to remove contributions to scattering from solvent molecules. The reported refinements are of guest-free structure by SQUEEZE routine. See Supplemetary Data 1 for further details. Transition metal ion exchange experiments Freshly prepared compound 1 (20 mg) was soaked in DMF solutions of nitrate salts of Cu 2+ , Co 2+ , Ni 2+ and Zn 2+ (5 ml, 0.1 mmol), respectively. After 5 days, the crystals were taken out of solution and washed with DMF to remove residual transition metal ions on the surface. The products were characterized by ICP and XRD and the results were listed in Supplementary Table S2 and Supplementary Fig. S6 . The photographs of the samples containing transition metal ions are presented in Supplementary Fig. S5 . Procedure for encapsulating [Ir(ppy) 2 (bpy)] + in 1 The samples of 1 (40 mg) were dipped in 10 ml DMF solutions containing 1 × 10 −4 mol L −1 [Ir(ppy) 2 (bpy)][PF 6 ] under stirring in 10 ml sealed glass bottles. After 0.5, 1, 2, 3, 4, 7 and 10 days, the immersed samples were taken out and washed with DMF to remove residual Ir complex on the surface. The concentrations of encapsulated [Ir(ppy) 2 (bpy)] + in [Ir(ppy) 2 (bpy)] + @ 1 were measured by ICP experiment and the results were shown in Supplementary Table S3 . The corresponding CIE coordinates were also calculated and listed in Supplementary Table S3 . Procedure for the preparation of lanthanide-doped compounds Eu/Tb@ 1 sample was prepared by immersing freshly prepared compound 1 in DMF solutions of lanthanide nitrates with molar ratios of 1:2 (total amount 0.03 mmol in 5 ml DMF). After 7 days of soakage, the crystals were taken out of solution and washed with DMF to remove residual lanthanide III cations on the surface. A similar process was employed to prepare Eu 3+ - or Tb 3+ -doped sample by soaking sample of 1 in DMF solutions of lanthanide nitrates of Eu 3+ or Tb 3+ (0.01 mmol in 5 ml DMF). After 5 and 7 days of soakage, respectively, the crystals were washed with DMF to remove residual lanthanide III cations on the surface. Fabrication of a simple WLED assembly A WLED was fabricated by dripping the white phosphor of 3.8 wt% [Ir(ppy) 2 (bpy)] + @ 1 on an ultraviolet InGaAsN LED chip ( λ ex =370 nm). The colour parameters of the device including CIE, CCT and CRI were measured by Ocean Optics USB 4000 Spectrometer at a forward current of 150 mA. Accession codes: The X-ray crystallographic coordinates for complex 1 have been deposited at the Cambridge Crystallographic Data Centre (CCDC), under deposition number CCDC 916964 . These data can be obtained free of charge from the Cambridge Crystallographic Data Centre via www.ccdc.cam.ac.uk/data_request/cif . How to cite this article: Sun, C-Y. et al. Efficient and tunable white-light emission of metal–organic frameworks by iridium-complex encapsulation. Nat. Commun. 4:2717 doi: 10.1038/ncomms3717 (2013).